Calcium-based multi-element chemistry for grid-scale electrochemical energy storage Calcium is an attractive material for the negative electrode in a rechargeable battery due to its low electronegativity (high cell voltage), double valence, earth abundance and low cost; however, the use of calcium has historically eluded researchers due to its high melting temperature, high reactivity and unfavorably high solubility in molten salts. Here we demonstrate a long-cycle-life calcium-metal-based rechargeable battery for grid-scale energy storage. By deploying a multi-cation binary electrolyte in concert with an alloyed negative electrode, calcium solubility in the electrolyte is suppressed and operating temperature is reduced. These chemical mitigation strategies also engage another element in energy storage reactions resulting in a multi-element battery. These initial results demonstrate how the synergistic effects of deploying multiple chemical mitigation strategies coupled with the relaxation of the requirement of a single itinerant ion can unlock calcium-based chemistries and produce a battery with enhanced performance. A liquid metal battery (LMB) consists entirely of liquid active components: a low-density liquid metal negative electrode, an intermediate-density molten salt electrolyte and a high-density liquid metal positive electrode. Due to their mutual immiscibility these active components further self-segregate into three distinct layers according to their densities. On discharge, the negative electrode is oxidized to form an itinerant ion, which migrates across the molten salt electrolyte to the positive electrode, where the itinerant ion is electrochemically reduced to neutral metal, alloying with the positive electrode. This process is reversed upon charging. The LMB is well-positioned to satisfy the demands of grid-scale energy storage due to its ability to vitiate capacity fade mechanisms present in other battery chemistries and to do so with earth abundant materials and easily scalable means of construction [1] , [2] . Owing to its high solubility in molten salts calcium is impractical as an electrode [1] , [3] , [4] . Metal solubility renders the molten salt electronically conductive [5] , which leads to loss of coulombic efficiency in electrolysis and loss of stored energy in a battery, that is, so-called self-discharge. In addition, the strong reducing capability of this electropositive element dispersed in the molten salt makes containment problematic, as most commonly used materials are susceptible to calciothermic reduction [6] . Herein we have made calcium the negative electrode of the LMB by devising parallel mitigation strategies to dramatically decrease its chemical potential so as to suppress both solubility and reactivity while advantageously lowering the melting temperature of the metal–salt couple. The detrimental dissolution reaction of calcium metal in calcium halides can be represented by the following [4] , [5] , [7] : where calcium metal (Ca) reacts with calcium cations (Ca 2+ ) to form subvalent ions (Ca + or ). Using the latter case as an example, the equilibrium constant of the dissolution reaction is therefore given as: where is the activity of dissolved subvalent calcium, a Ca the activity of calcium metal in negative electrode, and the activity of calcium cation in the electrolyte. Focusing on the contributions of the reactants, we reason that suppressing the activity of calcium metal in the negative electrode, a Ca , by alloying with more electronegative metals acting as diluents and that lowering the activity of Ca 2+ in the electrolyte, , by the introduction of other cations, should result in attendant reductions in the concentration of subvalent while simultaneously decreasing the reactivity and melting temperature of the negative electrode. It has been shown in our previous studies that alloying calcium with various positive electrodes drops the activity of calcium to values as low as 10 –9 (for bismuth) and 10 –10 (for antimony) [8] , [9] , indicative of strong chemical interactions. The low activity of calcium in these electrodes contributes to the high-cell voltage of calcium-based cells as well as to the suppression of calcium metal dissolution from the positive electrodes [3] . In previous work, we have confirmed the bi-directionality of these positive electrodes with coulombic efficiencies exceeding 99% for both calcium–bismuth (Ca–Bi) and calcium–antimony (Ca–Sb) [10] , [11] . Clearly, to obtain high-cell voltage, the activity of calcium in the negative electrode should be as high as possible. The challenge is how to suppress the solubility of calcium metal from the negative electrode without making it denser than the electrolyte or raising the melting point, while minimally reducing cell voltage. The present study shows that magnesium (Mg) is an effective diluent as it lowers the liquidus temperature of calcium–magnesium (Ca–Mg) alloy ( T eutectic =443 °C and 517 °C (ref. 12 )) while supporting adequate calcium activity over a wide range of composition [12] . Specifically, an electromotive force study of Ca–Mg alloys suggests that the cell voltage reduction can be minimized to <0.1 V as long as the calcium concentration remains above 30 mol% (ref. 12 ). Choosing the proper composition of multi-cation salts lowers the liquidus temperature of the electrolyte and decreases calcium solubility. The halides of the other cations in the multi-cation salt also work as supporting electrolytes, which desirably results in a lower ohmic drop under current flow. The choice of lithium chloride (LiCl) is advantageous due to its high ionic conductivity ( ∼ 4 S cm −1 ) [13] and its ability to form a low-melting eutectic mixture of lithium chloride and calcium chloride (LiCl–CaCl 2 , 65–35 mol%, T eutectic =485 °C (ref. 14 )). Furthermore, from the perspective of minimizing the self-discharge current, LiCl–CaCl 2 exhibited the best performance in the Ca–Mg||Bi cell. A liquid metal battery cell utilizing the Ca–Mg alloy as a negative electrode, the LiCl–CaCl 2 multi-cation mixture as an electrolyte, and a Bi positive electrode shows at 550 °C both high coulombic and energy efficiencies (>99% and >70%, respectively) and demonstrates no capacity fade in excess of 1,400 cycles. In addition, due to the similarity in the deposition potentials of lithium and calcium and their mutual solubility we have found that these two metals can jointly engage in charge-transfer reactions at both electrodes to establish a co-deposition energy storage device. Effects of electrode composition on cell performance A Ca–Mg (20–80 mol%)||Bi cell whose design is depicted in Fig. 1a was cycled at 200 mA cm −2 current density and 650 °C operating temperature. As shown in Fig. 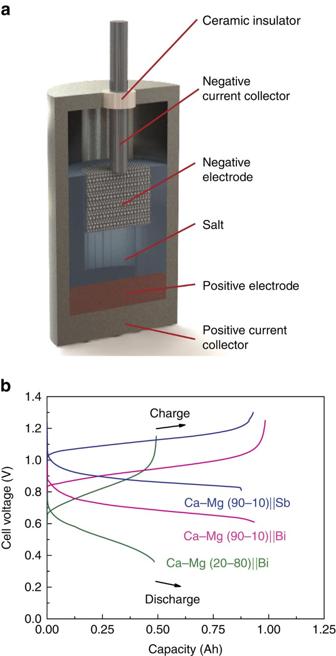Figure 1: Schematic and performance of Ca–Mg|LiCl–CaCl2|Bi and Sb cells. (a) Schematic of cell with the negative current collector consisting of a stainless steel rod and Fe–Ni foam and the positive current collector made of mild steel or graphite. The foam contains the negative electrode. Current collectors are electrically isolated by means of an alumina insulator. (b) Charge–discharge voltage time traces of Ca–Mg (20–80 mol%)||Bi, Ca–Mg (90–10 mol%)||Bi, and Ca–Mg (90–10 mol%)||Sb operated at current density 200 mA cm−2and temperature 650 °C. The theoretical capacities of Ca–Mg (20–80 mol%)||Bi, Ca–Mg (90–10 mol%)||Bi, and Ca–Mg (90–10 mol%)||Sb cells were 0.569, 1.33 and 1.08 Ah, respectively. The results of measurements were replicated more than five times, four times and twice, respectively. 1b the cell achieved 98% coulombic and 62% energy efficiencies with a discharge voltage of 0.52 V. The self-discharge current density of the cell, ∼ 1 mA cm −2 , is extremely low (see Supplementary Table 1 and Supplementary Note 1 ), comparable with that of the best-performing Li||Sb–Pb cells [2] . Even though the concentration of calcium in the negative electrode was quite low (20 mol%) the open-circuit voltage decreased only 0.18 V from that of a cell fitted with a pure calcium negative electrode [1] , [8] , [12] . 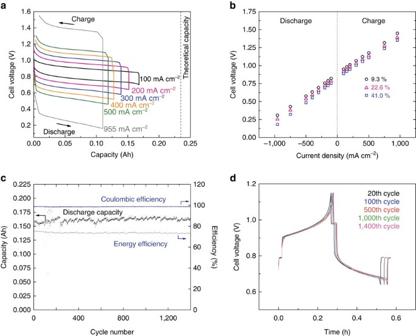Figure 2: Cell performance of Ca–Mg (90–10 mol%)||Bi cell. (a) Charge–discharge voltage time trace at current densities 100–955 mA cm−2. (b) Cell voltage with varying current density at 9.3, 22.6 and 41% of theoretical capacity. (c) Discharge capacity, coulombic efficiency and energy efficiency with cycling. (d) Representative charge–discharge voltage time traces at different cycle numbers. Theoretical capacity of this cell was 0.239 Ah. Operating temperature was 550 °C. Current density of (c,d) was 200 mA cm−2. The results derive from measurements on more than two cells. The volumetric energy density (electrodes basis) of this cell was 197 Wh L −1 (see Supplementary Table 2 ). In contrast, the higher calcium concentration Ca–Mg (90–10 mol%)||Bi cell maintained a cell-discharge voltage above 0.71 V and energy efficiency exceeding 70% ( Fig. 1b ). 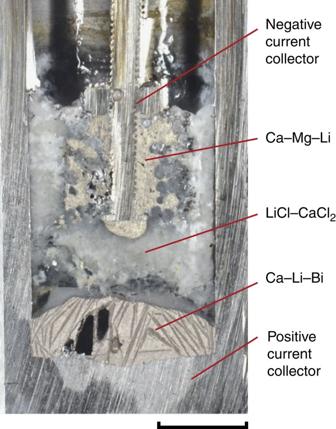Figure 3: Cross-section of Ca–Mg (90–10 mol%)||Bi cell at partial state of charge. The scale bar is 10 millimeter (mm). The results derive from measurements on more than three cells. The volumetric energy density of the cell increased to 329 Wh L −1 (see Supplementary Table 3 ). The high concentration of calcium in the negative electrode caused a slight reduction in coulombic efficiency to 96% as a result of a somewhat elevated self-discharge current density (≈4 mA cm −2 as shown in Supplementary Table 1 and Supplementary Note 1 ). This is well explained by the fact that at 600 °C the activity of calcium in magnesium is 2.9 × 10 −2 for 20–80 mol% Ca–Mg and ≈1 for 90–10 mol% Ca–Mg (ref. 12 ). Upon addition of 10 mol% of magnesium, the self-discharge current density was halved with almost no voltage penalty (≈0.01 V (refs 8 , 12 )) when compared with that of the pure Ca||Bi cell (≈ 10 mA cm −2 ). In sum, the Ca–Mg||Bi cells were designed to suppress the self-discharge current density while maintaining high cell voltage at a reduced operating temperature. In addition, a Ca–Mg negative electrode with a LiCl–CaCl 2 electrolyte can be operated with an antimony (Sb) positive electrode. With higher-cell voltage (0.88 V), higher energy efficiency (74%), and higher volumetric energy density (384 Wh L −1 , see Supplementary Table 4 ) the cell with an Sb positive electrode outperforms one with a Bi positive electrode as shown in Fig. 1b . Figure 1: Schematic and performance of Ca–Mg|LiCl–CaCl 2 |Bi and Sb cells. ( a ) Schematic of cell with the negative current collector consisting of a stainless steel rod and Fe–Ni foam and the positive current collector made of mild steel or graphite. The foam contains the negative electrode. Current collectors are electrically isolated by means of an alumina insulator. ( b ) Charge–discharge voltage time traces of Ca–Mg (20–80 mol%)||Bi, Ca–Mg (90–10 mol%)||Bi, and Ca–Mg (90–10 mol%)||Sb operated at current density 200 mA cm −2 and temperature 650 °C. The theoretical capacities of Ca–Mg (20–80 mol%)||Bi, Ca–Mg (90–10 mol%)||Bi, and Ca–Mg (90–10 mol%)||Sb cells were 0.569, 1.33 and 1.08 Ah, respectively. The results of measurements were replicated more than five times, four times and twice, respectively. Full size image Cell performance at lower operating temperature Exploiting the low eutectic temperatures of both the Ca–Mg alloy (90–10 mol%) and the binary LiCl–CaCl 2 electrolyte, we were able to decrease the cell operating temperature to 550 °C and obtain smooth voltage time traces at current densities ranging from 100 to 955 mA cm −2 ( Fig. 2a ). In parallel, the self-discharge current density of Ca–Mg (90–10 mol%)||Bi cells was found to decrease to <1 mA cm −2 ( Supplementary Fig. 1 ), which we attribute to the decrease in solubility of Ca in the electrolyte [4] , [7] , [15] . The fall in discharge capacity with increasing current density is a consequence of the fact that at high current densities the deposition rate of Ca at the electrode-electrolyte interface exceeds the rate of diffusion of Ca metal away from the electrode-electrolyte interface in the Bi positive electrode [10] , [11] . Because the theoretical capacity of the cell was defined as the mole fraction of calcium, at which the nucleation of the Ca 11 Bi 10 phase occurs (25 mol% at 550 °C (ref. 8 )), at high-current densities it is possible to reach this stoichiometry locally at the interface before the bulk metal electrode reaches this composition. The dependence of cell voltage on current density at several discharged states (9.3, 22.6 and 41.0% of theoretical capacity) is shown in Fig. 2b . The linearity in the I – V characteristic of the cell is evidence of the facile kinetics of the charge/discharge processes. This cell cycled at 200 mA cm −2 for over 1,400 cycles with 99% coulombic efficiency and 70% round-trip energy efficiency as depicted in Fig. 2c . The average volumetric energy density of this cell was 228 Wh L −1 (see Supplementary Table 5 ). Additionally noteworthy was that these metrics were achieved without observable voltage loss, side reactions or capacity fade as shown in Fig. 2c,d . Long service life-time translates to low cost of ownership, which is the most important parameter for grid-scale energy storage. No calcium metal battery has ever exhibited such stability. Figure 2: Cell performance of Ca–Mg (90–10 mol%)||Bi cell. ( a ) Charge–discharge voltage time trace at current densities 100–955 mA cm −2 . ( b ) Cell voltage with varying current density at 9.3, 22.6 and 41% of theoretical capacity. ( c ) Discharge capacity, coulombic efficiency and energy efficiency with cycling. ( d ) Representative charge–discharge voltage time traces at different cycle numbers. Theoretical capacity of this cell was 0.239 Ah. Operating temperature was 550 °C. Current density of ( c , d ) was 200 mA cm −2 . The results derive from measurements on more than two cells. Full size image Analysis of charge–discharge reactions Figure 3 shows the cross-section of a Ca–Mg (90–10 mol%)|| Bi cell in a partially discharged state. After 400 cycles at 550 °C, electrodes were subjected to chemical analysis by direct current plasma emission spectrometry. No corrosion was observed on either the negative or positive current collector. Significantly, both negative and positive electrodes in the partially discharged cells contain Li ( Supplementary Table 6 ). This means that both the Ca and Li ions in the multi-cation salt co-alloy and co-dealloy with both the negative and positive electrodes during charge and discharge. Furthermore, the absence of Mg in the positive electrode proves that there is no participation on the part of Mg in the cell electrochemistry, that is, Mg acts purely as a solvent to reduce the melting point of the negative electrode. The cell reactions can be represented as Figure 3: Cross-section of Ca–Mg (90–10 mol%)||Bi cell at partial state of charge. The scale bar is 10 millimeter (mm). The results derive from measurements on more than three cells. Full size image This unique multi-cation salt gives rise to the possibility of a multi-element LMB, in which a plurality of active metals participates in faradaic reactions. The high coulombic efficiency (>99%) and excellent retention of discharge capacity observed during lithium co-deposition indicate that the electrode reactions are fully bi-directional. Recognition that co-deposition in a battery can be managed to advantage broadens the selection of salt composition and extends the prediction of the capacity limit. This is in sharp contrast to the practice in calcium electrorefining which considers only those salts, for example, CaCl 2 –KCl, that obviate or suppress significant co-deposition to maintain the purity of the metal product [16] . The fact that this cell operates without need for an ion-selective membrane between the electrodes as is the case with sodium–sulfur and sodium–nickel chloride (ZEBRA) batteries, which rely on a β″-alumina separator, for example, sets this battery chemistry apart from all others. This membrane-free cell designed with a plurality of mitigation strategies opens up multi-element participation, which suppresses Ca reactivity, lowers operating temperature, and finally realizes a Ca-metal-based rechargeable battery that has the potential to meet the performance requirements of grid-scale energy storage applications. Cell configuration The negative current collector (NCC) consists of an 18–8 stainless steel threaded rod and a column-shaped Fe–Ni foam. The Fe–Ni foam was 13 mm in diameter, 10 mm in height, and 60 ppi in porosity. A mild steel (AISI 1018) crucible served as the positive current collector (PCC) for Bi. A graphite crucible served as the PCC for Sb. The dimensions of the PCCs were 25 mm in outer diameter, 83 mm in height, 77 mm in depth and 20 mm in inner diameter. The foam NCC was positioned 15 mm above the PCC. By surface tension the foam NCC holds the metal of the negative electrode and thus prevents keeps it from shorting to the positive current collector. The surface area of positive electrode was estimated at 3.14 cm 2 by assuming the interface between it and the electrolyte to be perfectly flat. This value was used to derive the current density. Materials preparation Pure Ca (99.99%, Aldrich), Mg (99.95%, Alfa Aesar), Bi (99.999%, Aldrich) and Sb (99.9999%, Alfa Aesar) were used for electrodes. These metals were melted in the PCCs by an induction heater (MTI Corporation, EQ-SP-15A), installed inside the glovebox with an inert argon atmosphere (O 2 <0.1 p.p.m., H 2 O<0.1 p.p.m.). Pure Ca and Mg were melted in a mild steel cup by the induction heater, and then the NCCs were immersed in the liquid Ca–Mg alloy for 10 min. High-purity anhydrous salts of LiCl (99.995%, Alfa Aesar) and CaCl 2 (99.99%, Alfa Aesar) were used. The salts were weighed out in appropriate quantities in ∼ 500 g batches, mixed, and transferred to an alumina crucible which was then placed in a stainless steel vacuum chamber, the chamber sealed, and loaded into a furnace. To prepare a dry, homogenous molten salt solution, the test chamber was (1) evacuated to ∼ 1 Pa, (2) heated at 80 °C for 12 h under vacuum, (3) heated at 230 °C for 12 h under vacuum, (4) purged with ultra-high-purity argon gas (99.999%, O 2 <1 p.p.m., H 2 O<1 p.p.m., Airgas Inc) and (5) heated at 700 °C for 3 h under argon gas flowing at 0.2 cm 3 s −1 . After cooling to room temperature, the pre-melted electrolyte was transferred back to the glove box and ground into powder (≈10 μm in diameter). Supplementary Table 7 reports the masses of metal and salt in each cell. To accelerate the measurement of long-term capacity fade at deep discharge (within several months instead of years), we reduced the size of the electrodes of the cell in Fig. 2 . It is important to restrict the depletion of LiCl so as to avoid solidification of the molten salt. According to the phase diagram of LiCl–CaCl 2 (ref. 14 ), at 550 °C for example, the liquid range of composition in the LiCl–CaCl 2 molten salt is 58–77 mol% of LiCl. To operate the cells at ∼ 1 Ah capacity we used ∼ 12 g of electrolyte thereby preventing solidification of the LiCl–CaCl 2 melt caused by depletion of LiCl via co-deposition of Li. Cell assembly Cells were loaded in the stainless steel vacuum chamber and subjected to the same drying process as were the salts (80 °C for 12 h and 230 °C for 12 h under vacuum). Then, the cells were connected to a battery tester (Model 4300, Maccor). The cells were heated under open circuit condition. After the temperature reached the liquidus of the electrolyte (485 °C), the cell voltage was held at 1.25 V until the current became steady. Analysis The measurement of self-discharge current density was performed after the cell reached the operating temperature and the current became steady at a constant applied voltage of 1.1 V reported in Supplementary Fig. 1 and of 1.25 V reported in Supplementary Table 1 . The charging and discharging voltage time traces were measured at constant current density. Data were acquired by battery testing instrumentation (Model 4300, Maccor). Coulombic efficiency ( η Q ) was calculated from charging capacity ( Q C ) and discharging capacity ( Q D ), . Energy efficiency ( η E ) was calculated from charging energy ( E C ) and discharging energy ( E D ), . Discharge voltage ( V D ) was calculated from discharge capacity and discharge energy ( V D =E D /Q D ). Theoretical discharge capacity of the cell was defined as the mole fraction of calcium, at which the nucleation of the Ca 11 Bi 10 phase occurs (25 mol% at 550 °C and 27 mol% at 650 °C (ref. 8 )) or the Ca 11 Sb 10 phase (23 mol% at 650 °C (ref. 11 )) assuming that only calcium participates in charge/discharge reaction. The volumetric energy density was calculated using the volumes of electrodes as shown in Supplementary Tables 2–5 . Direct-current plasma emission spectrometry was carried out by Luvak Inc., following ASTM E 1097–12. How to cite this article: Ouchi, T. et al . Calcium-based multi-element chemistry for grid-scale electrochemical energy storage. Nat. Commun. 7:10999 doi: 10.1038/ncomms10999 (2016).